Co-option of alternate sperm activation programs in the evolution of self-fertile nematodes Self-fertility evolved independently in three species of Caenorhabditi s, yet the underlying genetic changes remain unclear. This transition required that XX animals acquire the ability to produce sperm and then signal those sperm to activate and fertilise oocytes. Here, we show that all genes that regulate sperm activation in C. elegans are conserved throughout the genus, even in male/female species. By using gene editing, we show that C. elegans and C. briggsae hermaphrodites use the SPE-8 tyrosine kinase pathway to activate sperm, whereas C. tropicalis hermaphrodites use a TRY-5 serine protease pathway. Finally, our analysis of double mutants shows that these pathways were redundant in ancestral males. Thus, newly evolving hermaphrodites became self-fertile by co-opting either of the two redundant male programs. The existence of these alternatives helps explain the frequent origin of self-fertility in nematode lineages. This work also demonstrates that the new genome-editing techniques allow unprecedented power and precision in evolutionary studies. One of the major questions in evolutionary biology is how innovation occurs. Darwin [1] suggested that novel traits could be produced if older features were co-opted for new uses and subsequent research has confirmed this idea [2] . However, neither the qualities that determine which traits are co-opted to produce new features, nor the mechanisms that implement these changes are clear. For example, the genetic changes that led treehoppers to express a modified wing structure on the first thoracic segment [3] or beetles to produce a head horn [4] remain obscure. The origin of self-fertility in nematodes is ideal for tackling the problem [5] . Self-fertile hermaphrodites originated independently in three species of Caenorhabditis nematodes [6] , [7] , [8] ( Fig. 1a ). This step required XX animals to acquire the ability to (1) produce sperm and (2) signal those sperm to activate and fertilise oocytes [9] . As these transitions occurred recently, it might be possible to identify the underlying changes by comparative analysis. 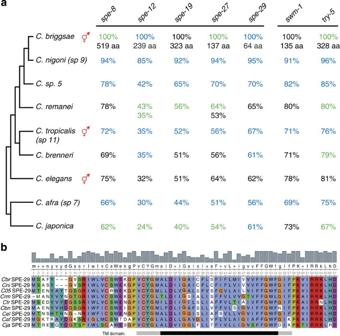Figure 1: All sperm activation genes are conserved throughoutCaenorhabditis. (a) Percent identity of each protein to itsC. briggsaeortholog. In the phylogeny8at left, each androdioecious species is marked in red. Percentages for newly described proteins are blue and for revised proteins are green.C. remaneihas duplicates ofspe-12andspe-27.(b) Representative alignment of SPE-29 sequences, prepared using MUSCLE45. A conserved transmembrane domain is marked with the core in black and variable edges in grey46. For brevity,C. sp. 5has been abbreviatedC05in the figure. Figure 1: All sperm activation genes are conserved throughout Caenorhabditis. ( a ) Percent identity of each protein to its C. briggsae ortholog. In the phylogeny [8] at left, each androdioecious species is marked in red. Percentages for newly described proteins are blue and for revised proteins are green. C. remanei has duplicates of spe-12 and spe-27. ( b ) Representative alignment of SPE-29 sequences, prepared using MUSCLE [45] . A conserved transmembrane domain is marked with the core in black and variable edges in grey [46] . For brevity, C. sp. 5 has been abbreviated C05 in the figure. Full size image Studies with C. elegans showed that five genes are required to initiate hermaphrodite sperm activation in that species— spe-8 (refs 10 , 11 ), spe-12 (refs 10 , 12 ), spe-19 (ref. 13 ), spe-27 (ref. 14 ) and spe-29 (ref. 15 ). Mutations in any of these genes block hermaphrodite self-fertility, but do not prevent male sperm from activating and fertilising oocytes. All five genes are expressed in sperm and three encode transmembrane proteins [16] . Furthermore, SPE-8 is a protein tyrosine kinase whose localisation to the plasma membrane in spermatids requires the other genes [11] . Thus, these five proteins might define a complex located on the plasma membrane that responds to an extracellular signal controlling activation. Although one candidate for this signal is extracellular zinc [17] , none of the proteins from the SPE-8 group has known zinc-binding domains or zinc importation motifs. Recently, the TRY-5 protease was shown to act in a second sperm activation pathway, which functions only in males [18] , [19] . Before mating, TRY-5 activity is inhibited by SWM-1, a protein with two trypsin inhibitor-like domains [20] . During ejaculation, large TRY-5 reserves are secreted into the seminal fluid, where they activate male spermatids. Although their direct target is unknown, one possibility is SNF-10, a membrane protein found in sperm [21] . Although try-5 males are fertile, the spe-8; try-5 double mutants are sterile, which indicates that these two signal transduction pathways are redundant in C. elegans [18] . However, special mutations in spe-6 (ref. 22 ), spe-4 (ref. 23 ) and spe-46 (ref. 24 ), which are all required for spermatogenesis, can bypass the need for these signals in the activation process. For example, spe-6(hc163) is epistatic to both try-5 (ref. 18 ) and spe-8 (ref. 22 ), so the SPE-6 kinase probably acts within spermatids to respond to extracellular signals and cause activation. Intra-species crosses showed that some aspects of sperm activation are conserved in Caenorhabditis, although the molecular details remain unknown [25] . As experimental studies using C. remanei revealed that female nematodes lack a mechanism to activate sperm [9] , learning which methods of sperm activation are used by hermaphrodites from diverse species is critical for understanding the origins of self-fertility. Here, we show that two redundant sperm activation pathways have been conserved in Caenorhabditis. Hermaphrodites from C. elegans and C. briggsae require the SPE-8 pathway to activate their sperm, whereas hermaphrodites from C. tropicalis require the TRY-5 pathway. The ability to co-opt either of two alternative signal transduction pathways could explain the frequent origin of self-fertility in this group of animals. Sperm activation genes are conserved in Caenorhabditis To begin, we identified orthologs of all C. elegans sperm activation genes in the eight-related species for which partial genome sequences were available. Previously, only 23 of these sperm activation genes had been identified. Using BLAST searches and phylogenetic comparisons, we refined these predictions and identified the remaining 33 genes ( Fig. 1 , Supplementary Fig. 1 ). We used degenerate oligonucleotides to clone Cbr-spe-12, which was missing from the genome assembly, and the PCR to isolate missing parts of Ctr-spe-8 and Ctr-spe-27 . Our results show that the ancestor of Caenorhabditis had orthologs of all seven sperm activation genes. Moreover, each of the encoded proteins has conserved elements, like the transmembrane domain of SPE-29 ( Fig. 1b ) or the kinase domain of SPE-8. As the common ancestor and six species are male/female, none of these genes is likely to function exclusively in hermaphrodites. We used reverse transcription PCR (RT–PCR) to characterise the expression of each gene in C. briggsae. The five members of the C. elegans spe-8 group are expressed in spermatids [16] , where they respond to an unknown signal. In C. briggsae, their expression is also correlated with spermatogenesis—the transcripts are present in larval hermaphrodites, larval males and adult males, but absent from adult hermaphrodites ( Fig. 2a and Supplementary Fig. 2 ). Thus, genes of the spe-8 group appear to produce sperm proteins in C. briggsae, as they do in C. elegans. By contrast, C. briggsae try-5 and swm-1 transcripts were detected in all animals, including adult hermaphrodites. 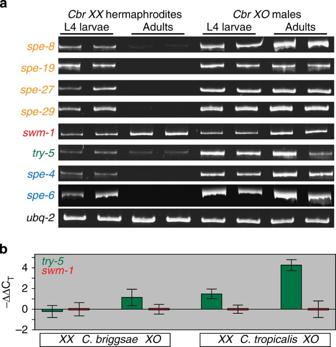Figure 2: Sperm activation genes are expressed in males and some hermaphrodites. (a) Semi-quantitative RT–PCR analysis of RNA from independent samples of each indicated age and sex. The genesspe-4andspe-6were control spermatogenesis genes and the ubiquitin geneubq-2was a loading control. (b) Real-time RT–PCR analysis of the indicated genes and animals at the L4 larval stage. There were three biological replicates of each sample, each of which had two technical replicates; the error bars represent standard error of the mean. Note thattry-5levels are higher relative toswm-1levels in the three groups that use TRY-5 to activate sperm, but not inC. briggsaehermaphrodites, which instead use thespe-8pathway. Figure 2: Sperm activation genes are expressed in males and some hermaphrodites. ( a ) Semi-quantitative RT–PCR analysis of RNA from independent samples of each indicated age and sex. The genes spe-4 and spe-6 were control spermatogenesis genes and the ubiquitin gene ubq-2 was a loading control. ( b ) Real-time RT–PCR analysis of the indicated genes and animals at the L4 larval stage. There were three biological replicates of each sample, each of which had two technical replicates; the error bars represent standard error of the mean. Note that try-5 levels are higher relative to swm-1 levels in the three groups that use TRY-5 to activate sperm, but not in C. briggsae hermaphrodites, which instead use the spe-8 pathway. Full size image The SPE-8 group regulates XX sperm activation in C. briggsae To learn how these genes functioned, we used TALENs to generate knockout mutants of key members of the spe-8 group in C. briggsae [26] , [27] , [28] ( Fig. 3a ). We found that mutations in Cbr-spe-8 and Cbr-spe-19 caused XX animals to produce inactive spermatids ( Fig. 3b ), which prevented self-fertility ( Fig. 3c ). This effect was strongest for frame-shifting alleles, which are probably null, and more mild for Cbr-spe-19(v173), which inserts six amino acids. Because the C. briggsae mutant males were fertile, all of these strains could be maintained as male/hermaphrodite populations, so the mutant oocytes function normally. In addition, some sperm in these mutant hermaphrodites could be transactivated by seminal fluid from males, restoring self-fertility ( Fig. 3d ). This entire suite of phenotypes resembles that of their C. elegans counterparts [10] , [13] . 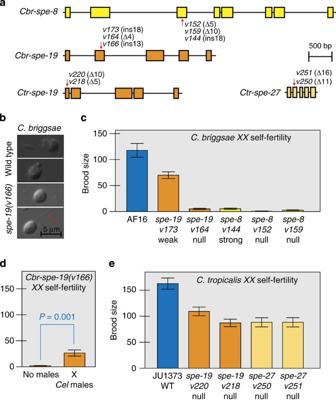Figure 3: Thespe-8group controls hermaphrodite sperm activation inC. briggsaebut notC. tropicalis. (a) Gene structures. Each 5′ end is left and exons are boxed. Mutation sites are indicated with arrows. (b) Sperm isolated fromC. briggsaewild-type hermaphrodites were active, and those fromspe-19(v166)were inactive or had only spiky protrusions (red arrow). (c) Thespe-8group is required for sperm activation inC. briggsaehermaphrodites. Brood size is the number of eggs laid by unmated hermaphrodites of each genotype. Bars show standard error of the mean. (d)C. briggsae spe-19sperm can be transactivated by male seminal fluid. We usedC. elegans fog-2males, which cannot fertiliseC. briggsae47. The significance was determined with a Student’st-test. (e) Thespe-8group is not required for hermaphrodite sperm activation inC. tropicalis. Figure 3: The spe-8 group controls hermaphrodite sperm activation in C. briggsae but not C. tropicalis. ( a ) Gene structures. Each 5′ end is left and exons are boxed. Mutation sites are indicated with arrows. ( b ) Sperm isolated from C. briggsae wild-type hermaphrodites were active, and those from spe-19(v166) were inactive or had only spiky protrusions (red arrow). ( c ) The spe-8 group is required for sperm activation in C. briggsae hermaphrodites. Brood size is the number of eggs laid by unmated hermaphrodites of each genotype. Bars show standard error of the mean. ( d ) C. briggsae spe-19 sperm can be transactivated by male seminal fluid. We used C. elegans fog-2 males, which cannot fertilise C. briggsae [47] . The significance was determined with a Student’s t -test. ( e ) The spe-8 group is not required for hermaphrodite sperm activation in C. tropicalis. Full size image As the spe-8 group of genes predated the origin of self-fertility, we wondered if the similarity between C. elegans and C. briggsae was caused by chance or a developmental bias [29] that favoured the use of these genes in hermaphrodites. Thus, we examined a third androdioecious species— C. tropicalis (formerly sp. 11) (refs 8 , 30 ). Null alleles in Ctr-spe-19 and Ctr-spe-27 had only a mild effect on reproduction, and the mutant hermaphrodites were all self-fertile ( Fig. 3e ). Thus, the spe-8 group is required for hermaphrodite sperm activation in C. elegans and C. briggsae , but not in C. tropicalis. Another pathway must activate sperm in hermaphrodites of that species. TRY-5 regulates XX sperm activation in C. tropicalis Next, we studied the try-5 pathway, which regulates sperm activation in C. elegans [18] and A. suum [19] males. TRY-5 is a trypsin protease that cleaves an unknown target on the surface of sperm. In C. elegans, TRY-5 is secreted by the male gonad, and its activity is blocked by the protease inhibitor SWM-1, preventing premature activation [20] . We found that knocking out swm-1 caused male sperm to activate prematurely in both C. briggsae ( Fig. 4a,b ) and C. tropicalis ( Fig. 5a ). These results show that the role of SWM-1 has been conserved. Null alleles of C. briggsae try-5 had no phenotype on their own, but did suppress swm-1 mutations ( Fig. 4a,b ), implying that Cbr- SWM-1 works through TRY-5 to control activation ( Fig. 4c ). Similarly, knocking down try-5 activity in C. tropicalis suppressed the premature activation caused by swm-1 mutations in that species ( Fig. 5a,b ). These phenotypes all resemble those seen in C. elegans [18] , [20] . However, we were surprised to find that Ctr-try-5 males were infertile, so the spe-8 group of genes is not sufficient for sperm activation in males of this species ( Fig. 5c ). 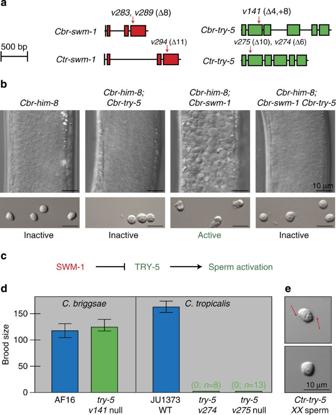Figure 4: TRY-5 controls sperm activation in males andC. tropicalishermaphrodites. (a) Gene structures. Each 5′ end is left and exons are boxed. Mutation sites are indicated with arrows. (b) Differential interference contrast photomicrogaphs of gonads fromC. briggsaemales 1 day after the L4 larval stage (above) and sperm from dissected males (below). Scale bars, 10 μm. (c) Summary of the results of genetic epistasis. Theswm-1gene must act throughtry-5to regulate male sperm activation, as it does inC. elegans18,20. (d) TRY-5 is absolutely required for self-fertility inC. tropicalishermaphrodites, but not inC. briggsaeones. (e) Spermatids isolated fromCtr-try-5(v275)hermaphrodites have not been activated, although some have spiky projections (red arrows). Figure 4: TRY-5 controls sperm activation in males and C. tropicalis hermaphrodites. ( a ) Gene structures. Each 5′ end is left and exons are boxed. Mutation sites are indicated with arrows. ( b ) Differential interference contrast photomicrogaphs of gonads from C. briggsae males 1 day after the L4 larval stage (above) and sperm from dissected males (below). Scale bars, 10 μm. ( c ) Summary of the results of genetic epistasis. The swm-1 gene must act through try-5 to regulate male sperm activation, as it does in C. elegans [18] , [20] . ( d ) TRY-5 is absolutely required for self-fertility in C. tropicalis hermaphrodites, but not in C. briggsae ones. ( e ) Spermatids isolated from Ctr-try-5(v275) hermaphrodites have not been activated, although some have spiky projections (red arrows). 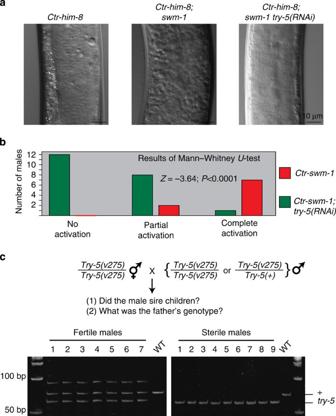Figure 5:C. tropicalisTRY-5 is required for male fertility. (a) Photomicrographs of adult males of the indicated genotypes, scored 2 days after the L4 larval stage. Thectr-swm-1(v294)mutation causes male sperm to activate before ejaculation, resulting in a characteristic rough appearance. This activation depends on TRY-5, because it is suppressed by knocking downtry-5with RNAi, (using 2.4 μg μl−1double-stranded RNA). (b) Histogram showing the extent of sperm activation inC. tropicalismales that were eitherhim-8; swm-1(v294)orhim-8; swm-1(v294); try-5(RNAi). (c) Results of individual crosses betweenCtr-try-5mothers and single males that were either homozygous or heterozygous fortry-5.After mating had occurred (as judged by the presence of a plug), the plates were scored for progeny and the P0males were removed for PCR analysis. All fertile males were heterozygotes and all sterile males weretry-5homozygotes. The upper band is a byproduct of the PCR reaction found in animals heterozygous for these two alleles. Full size image Figure 5: C. tropicalis TRY-5 is required for male fertility. ( a ) Photomicrographs of adult males of the indicated genotypes, scored 2 days after the L4 larval stage. The ctr-swm-1(v294) mutation causes male sperm to activate before ejaculation, resulting in a characteristic rough appearance. This activation depends on TRY-5, because it is suppressed by knocking down try-5 with RNAi, (using 2.4 μg μl −1 double-stranded RNA). ( b ) Histogram showing the extent of sperm activation in C. tropicalis males that were either him-8; swm-1(v294) or him-8; swm-1(v294); try-5(RNAi) . ( c ) Results of individual crosses between Ctr-try-5 mothers and single males that were either homozygous or heterozygous for try-5. After mating had occurred (as judged by the presence of a plug), the plates were scored for progeny and the P 0 males were removed for PCR analysis. All fertile males were heterozygotes and all sterile males were try-5 homozygotes. The upper band is a byproduct of the PCR reaction found in animals heterozygous for these two alleles. Full size image When we examined hermaphrodites, we found that C. tropicalis try-5 mutations blocked self-fertility, whereas C. briggsae try-5 mutations had no effect ( Fig. 4d ). Sterile Ctr-try-5 hermaphrodites produced normal oocytes, because they made cross progeny when fertilised by males. However, some sperm were completely inactive and others had spiky projections rather than pseudopods, which might indicate defective activation ( Fig. 4e ). Thus, TRY-5 is required for sperm activation in C. tropicalis hermaphrodites, whereas the spe-8 group is essential in C. elegans and C. briggsae hermaphrodites. As one might expect given this result, try-5 expression in C. tropicalis hermaphrodites is high relative to that of swm-1 ( Fig. 2b ). SPE-8 and TRY-5 pathways were redundant in ancestral males To learn how these differences originated, we studied C. briggsae males. These experiments were motivated by genetic tests showing that the TRY-5 and SPE-8 pathways are redundant in C. elegans males [18] . We found that Cbr-try-5 males produced numerous progeny when crossed with Cbr-try-5 spe-19 hermaphrodites, but that Cbr-try-5 spe-19 males produced few or none ( Fig. 6a ). This decrease in male fertility shows that these sperm activation pathways are redundant in C. briggsae . Given the phylogeny, this result implies that the common ancestor was a male/female species that used both pathways to activate male sperm ( Fig. 6b ). 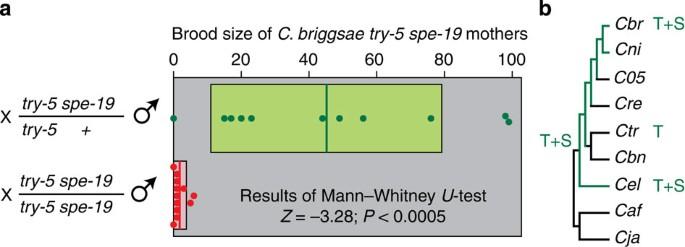Figure 6: The TRY-5 and SPE-8 pathways were redundant in ancestral males. (a) Analysis of crosses testing the fertility ofCbr-try-5(v141)males that were heterozygous or homozygous forspe-19(v166).We selected individual non-Unc male progeny fromhim-8; try-5+unc-51/ try-5 spe-19+mothers. After each male was crossed with atry-5 spe-19sterile mother, its genotype was determined by the PCR. Successful crosses were identified by mating plugs and scored for offspring the following day. Statistical calculations were done usingvassarstats.net/utest.html. (b) Phylogeny of theelegansgroup, showing male sperm activation pathways (T=TRY-5 and S=SPE-8 group). On the basis of parsimony, ancestral males used both the TRY-5 and SPE-8 pathways. Figure 6: The TRY-5 and SPE-8 pathways were redundant in ancestral males. ( a ) Analysis of crosses testing the fertility of Cbr-try-5(v141) males that were heterozygous or homozygous for spe-19(v166). We selected individual non-Unc male progeny from him-8; try-5+unc-51/ try-5 spe-19+ mothers. After each male was crossed with a try-5 spe-19 sterile mother, its genotype was determined by the PCR. Successful crosses were identified by mating plugs and scored for offspring the following day. Statistical calculations were done using vassarstats.net/utest.html . ( b ) Phylogeny of the elegans group, showing male sperm activation pathways (T=TRY-5 and S=SPE-8 group). On the basis of parsimony, ancestral males used both the TRY-5 and SPE-8 pathways. Full size image Why have these redundant pathways been conserved? Studies of C. elegans showed that some mutants in the spe-8 group decreased male fertility, so these genes might control additional aspects of sperm function [12] , [15] . When we tested Cbr-spe-19 and Ctr-spe-19 males by crossing them with hermaphrodites, we found that their sperm activated but competed poorly for fertilisation ( Fig. 7 and Supplementary Fig. 3 ). Thus, these redundant activation pathways may have persisted because they have additional, non-overlapping functions. However, in C. tropicalis , the overlap between these activation pathways is minimal, as the ctr-try-5 males are sterile ( Fig. 5c ). Thus, it is possible that the functions of the SPE-8 and TRY-5 systems are diverging in this species. 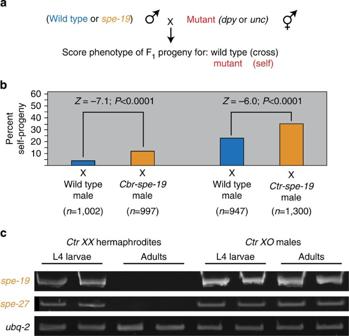Figure 7: Thespe-19gene helps produce optimal sperm inC. briggsaeandC. tropicalis. (a) Method for measuring the ability of male sperm to compete with hermaphrodite sperm. After a brief mating, the progeny were counted for several days. To ensure that male-derived sperm were present during scoring, all data were from intermediate days, which were both preceded and followed by days with cross progeny. The mutations werecbr-spe-19(v166)orctr-spe-19(v218)and the markers werecbr-dpy-11orctr-unc-23.(b) The significance of the difference between the pairs of proportions was calculated atvassarstats.net/propdiff_ind.html. (c) Semi-quantitative RT–PCR analysis of RNA from independent samples of each indicated age and sex reveals thatC. tropicalismales express genes of thespe-8group. The ubiquitin geneubq-2was a loading control. Figure 7: The spe-19 gene helps produce optimal sperm in C. briggsae and C. tropicalis . ( a ) Method for measuring the ability of male sperm to compete with hermaphrodite sperm. After a brief mating, the progeny were counted for several days. To ensure that male-derived sperm were present during scoring, all data were from intermediate days, which were both preceded and followed by days with cross progeny. The mutations were cbr-spe-19(v166) or ctr-spe-19(v218) and the markers were cbr-dpy-11 or ctr-unc-23. ( b ) The significance of the difference between the pairs of proportions was calculated at vassarstats.net/propdiff_ind.html . ( c ) Semi-quantitative RT–PCR analysis of RNA from independent samples of each indicated age and sex reveals that C. tropicalis males express genes of the spe-8 group. The ubiquitin gene ubq-2 was a loading control. Full size image The sister species to C. briggsae lacks XX sperm activation Our data suggested that XX animals co-opt one of the male sperm activation systems during the evolution of self-fertility. However, this model rests on the idea that females in gonochoristic species do not use sperm activations signals, which previously had been tested only in C. remanei [9] . Thus, we carried out similar experiments with the gonochoristic species C. nigoni, which is so closely related to C. briggsae that the two can mate and produce fertile offspring [8] , [31] . We found that C. nigoni XX animals that were induced to produce spermatids, as well as oocytes by RNA interference (RNAi) were not self-fertile ( Fig. 8a ), just as observed with C. remanei . However, when we induced C. nigoni/C. briggsae hybrids to produce spermatids, their sperm activated and the animals made self-progeny ( Fig. 8c ). Thus, C. briggsae produces a dominant factor that activates sperm in XX animals, but C. nigoni lacks this factor. 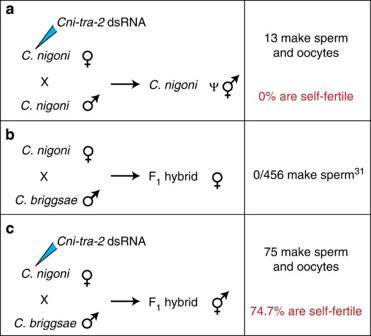Figure 8:C. briggsaecontains a dominant gene that can activate sperm. (a)C. nigoni tra-2(RNAi) XXanimals can develop as pseudohermaphrodites, just as those observed inC. remanei9. Out of 109 F1XXprogeny we observed 54 females, 13 pseudohermaphrodites and 42 Mog animals (which produced only sperm but had female bodies). The pseudohermaphrodites were not self-fertile and their sperm did not appear to have activated. (b)C. briggsaeandC. nigoniare sister species that produce fertile female progeny; these hybrid animals do not make sperm31. (c) Whentra-2activity was knocked down by RNAi in the hybrid progeny (using 1 μg μl−1double-stranded RNA), most of the animals that produced sperm were self-fertile. Out of 119 F1XXprogeny we observed 56 self-fertile hermaphrodites but only 19 animals that laid oocytes and did not lay eggs, which implies that they produced inactive sperm. This result shows thatC. briggsaecontains a dominant factor that activates sperm, which is consistent with models in whichC. briggsaehermaphrodites secrete an activating signal. Figure 8: C. briggsae contains a dominant gene that can activate sperm. ( a ) C. nigoni tra-2(RNAi) XX animals can develop as pseudohermaphrodites, just as those observed in C. remanei [9] . Out of 109 F 1 XX progeny we observed 54 females, 13 pseudohermaphrodites and 42 Mog animals (which produced only sperm but had female bodies). The pseudohermaphrodites were not self-fertile and their sperm did not appear to have activated. ( b ) C. briggsae and C. nigoni are sister species that produce fertile female progeny; these hybrid animals do not make sperm [31] . ( c ) When tra-2 activity was knocked down by RNAi in the hybrid progeny (using 1 μg μl −1 double-stranded RNA), most of the animals that produced sperm were self-fertile. Out of 119 F 1 XX progeny we observed 56 self-fertile hermaphrodites but only 19 animals that laid oocytes and did not lay eggs, which implies that they produced inactive sperm. This result shows that C. briggsae contains a dominant factor that activates sperm, which is consistent with models in which C. briggsae hermaphrodites secrete an activating signal. Full size image These results point to a simple model for the origin of self-fertility in hermaphroditic nematodes. The ancestor of the elegans group was a male/female species [6] , [7] , [8] , and the males used two redundant signals to activate sperm ( Fig. 9a ), whereas the females did not produce either signal [9] ( Fig. 9b ). When C. elegans, C. tropicalis and C. briggsae began the transformation to self-fertility, the XX animals co-opted one or the other of the male pathways ( Fig. 9c,d ), but did not need both. As predicted by this model, C. briggsae contains a dominant factor that can activate sperm in intra-species hybrids. 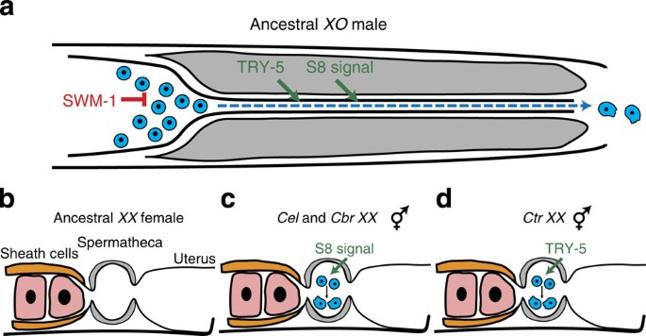Figure 9: The TRY-5 and SPE-8 pathways were redundant in ancestral males. (a) Model showing redundant sperm activation signals in ancestral males. These signals were produced in the somatic gonad and released in seminal fluid during ejaculation. S8 signal=unknown signal that acts on the SPE-8 group. (b–d)C. elegansandC. briggsaehermaphrodites co-opted the S8 signal to become self-fertile, butC. tropicalishermaphrodites co-opted TRY-5. Figure 9: The TRY-5 and SPE-8 pathways were redundant in ancestral males. ( a ) Model showing redundant sperm activation signals in ancestral males. These signals were produced in the somatic gonad and released in seminal fluid during ejaculation. S8 signal=unknown signal that acts on the SPE-8 group. ( b – d ) C. elegans and C. briggsae hermaphrodites co-opted the S8 signal to become self-fertile, but C. tropicalis hermaphrodites co-opted TRY-5. Full size image The ability to co-opt specific genetic programs might underlie the origin of many complex traits [32] and could explain some examples of parallel evolution [33] . Our data strongly support this model, as we show that nematodes have co-opted male sperm activation programs for use in newly evolving hermaphrodites. More importantly, we found that two different sperm activation programs can be co-opted for this purpose. Usually, developmental biases or constraints are thought to prevent certain types of variation from occurring, which prevents some evolutionary transitions [29] . Our results imply that some patterns of developmental regulation favour certain types of change, as the existence of two sperm activation pathways in nematodes helps explain why self-fertility has originated so frequently in this group [8] . Thus, this system provides a concrete example of the concept of evolvability in evolutionary developmental biology [34] . Although cases of convergent or parallel evolution provide natural experiments that illuminate evolutionary processes, their definitions remain controversial [35] , [36] . Usually, they are thought of as distinct phenomena—parallel evolution occurs through the independent origin and fixation of mutations affecting the same gene, whereas convergence occurs when selection leads to different solutions to the same problem. Our results show that this distinction is often artificial, as the two Caenorhabditis species evolved self-fertility by recruiting the spe-8 pathway to control hermaphrodite sperm activation (parallel evolution) but a third achieved the same end by recruiting the try-5 pathway (convergent evolution). Finally, our work shows that entire pathways in newly described species can be subjected to precise evolutionary genetic comparisons through gene editing. Although RNAi has been invaluable for evolutionary studies, phenotypes often vary between species because of differential sensitivity to RNAi [37] , rather than because the targeted pathways have changed. Even more problematic, some phenotypes (like those of nematode sperm) are often recalcitrant to RNAi. By contrast, gene editing using TALENs [26] , [27] , [28] or CRISPRs [38] , [39] can produce comparable alleles in each species. As these mutations allow rigorous comparisons of phenotype, we anticipate that their use will soon become routine. Strains and genetics C. briggsae mutants were derived from the wild isolate AF16 (ref. 40 ). They include: LG I : him-8(v188) (ref. 28 ); LGIV: she-1(v49) (ref. 41 ); LGV: dpy-11(v241) (ref. 28 ), unc-51(v205) (ref. 28 ) and new mutations described in the manuscript. C. nigoni RNAi experiments were done using JU1421 (M. Felix, pers. comm.). C. tropicalis mutants were derived from the wild isolate JU1373 (ref. 8 ). They include unc-23(v277) (ref. 28 ), him-8(v287), which deletes 9 nt and adds 4 nt, and those described in the figures. Cloning and sequencing To identify the C. briggsae spe-12 gene, we used degenerate nucleotides designed according to the CODE-HOP protocol [42] . Missing portions of Ctr-spe-8 and C. sp. 5 spe-27 were amplified from genomic DNA using flanking primers. PCR products were purified with a PCR Purification kit (Qiagen) and sequenced (GeneWiz). Primers are listed in Supplementary Table 1 . RNA interference Templates were amplified from mixed stage complementary DNA or genomic DNA by the PCR, with primers that contained a T7 promoter ( Supplementary Table 1 ), purified with a PCR Purification kit (Qiagen) and transcribed using MegaScript (Ambion). After annealing, double-stranded RNA was purified with MegaClear (Ambion). RNAi was performed by injection [43] . Semi-quantitative RT–PCR Groups of five worms of the desired age and sex were collected and processed as described [44] ; two independent samples were prepared to confirm reproducibility. RT–PCR was carried out using HotMaster Taq DNA polymerase (5PRIME) and MMLV Reverse Transcriptase (Invitrogen). PCR reactions were run for 35 cycles using primers from Supplementary Table 1 . Real-time quantitative RT–PCR Groups of five worms of the desired age and sex were prepared as described above; at least three independent biological replicates and two technical replicates were assayed for each data point. For each reaction, 1/20 of the total complementary DNA sample was used in a final volume of 25 μl, which included 12.5 μl of FastStart Universal SYBR Green Master (Rox, Roche) and 6 μM primers ( Supplementary Table 1 ). Amplification was 40 cycles, using Applied Biosystems 7500 Real-Time PCR Systems. Samples that did not show detectable amplification by the final cycle were arbitrarily assigned a Ct value of 40. The ΔCt values for swm-1 and try-5 were calculated for each group of L4 larvae, and normalised to control ubq-2 transcript levels. Afterwards, −ΔΔCt values were calculated for each group by comparing transcript levels for each sex and species with the corresponding swm-1 levels for those animals. Error bars are based on standard error of the mean. Microscopy Sperm were isolated as described [9] . Whole worms and isolated sperm were observed with differential interference contrast microscopy. Images were captured with a Zeiss Axiocam digital camera and Zeiss AxioVision software and assembled using Adobe Photoshop. TALEN knockout mutants TALENs were designed and produced as described [28] ( Supplementary Table 2 ). To create mutants, pairs of TALEN messenger RNAs were injected into the gonads of adult hermaphrodites [26] . At 20 °C, the F 1 progeny from a 6 to 32 h time window were singled to new plates at the L4 stage, and those F 1 animals that carried new mutations were identified by phenotype or by PCR analysis of the target site (primers in Supplementary Table 1 ). Fertility assays To assess hermaphrodite fertility, individual L4 animals were singled and transferred daily to new plates. After the mother was removed, each plate was scored by inspection for the number of progeny. Male fertility was assayed similarly, after crosses between single males and single females or hermaphrodites. How to cite this article: Wei, Q. et al. Co-option of alternate sperm activation programs in the evolution of self-fertile nematodes. Nat. Commun. 5:5888 doi: 10.1038/ncomms6888 (2014). Accession codes: The C. briggsae spe-12 sequence has been deposited in the GenBank database with accession code KP123338 .